Structure–function characterization reveals new catalytic diversity in the galactose oxidase and glyoxal oxidase family Alcohol oxidases, including carbohydrate oxidases, have a long history of research that has generated fundamental biological understanding and biotechnological applications. Despite a long history of study, the galactose 6-oxidase/glyoxal oxidase family of mononuclear copper-radical oxidases, Auxiliary Activity Family 5 (AA5), is currently represented by only very few characterized members. Here we report the recombinant production and detailed structure–function analyses of two homologues from the phytopathogenic fungi Colletotrichum graminicola and C. gloeosporioides , Cgr AlcOx and Cgl AlcOx, respectively, to explore the wider biocatalytic potential in AA5. EPR spectroscopy and crystallographic analysis confirm a common active-site structure vis-à-vis the archetypal galactose 6-oxidase from Fusarium graminearum . Strikingly, however, Cgr AlcOx and Cgl AlcOx are essentially incapable of oxidizing galactose and galactosides, but instead efficiently catalyse the oxidation of diverse aliphatic alcohols. The results highlight the significant potential of prospecting the evolutionary diversity of AA5 to reveal novel enzyme specificities, thereby informing both biology and applications. The enzyme-catalysed oxidation of diverse aliphatic and aromatic alcohols is a ubiquitous reaction in nature that is central to many biological processes and which forms the basis for a range of biotechnological applications [1] , [2] , [3] , [4] , [5] , [6] . Within the Enzyme Commission classification, alcohol oxidoreductases are primarily distinguished by the electron acceptor substrate, with the NAD + /NADP + -dependent ‘alcohol dehydrogenases’ (EC 1.1.1) constituting the historically richest, largest and most diverse class [1] , [7] (see also http://www.chem.qmul.ac.uk/iubmb/enzyme/EC1/1/1/ ). Enzymes from the second most diverse class of alcohol oxidoreductases, traditionally known as ‘alcohol oxidases (AOX)’, employ molecular oxygen as a terminal electron acceptor to generate hydrogen peroxide (EC 1.1.3). Many of these enzymes are flavoproteins that are dependent on the FAD + cofactor as an initial electron acceptor [1] , [6] . EC 1.1.3 also comprises non-FAD + -dependent enzymes, including copper-radical oxidases (CROs) such as glyoxal oxidases (EC 1.1.3.-), hexose 1-oxidases (EC 1.1.3.5) and galactose 6-oxidases (EC 1.1.3.9; refs 6 , 8 , see also http://www.chem.qmul.ac.uk/iubmb/enzyme/EC1/1/3/ ). Owing to their lack of dependence on an organic cofactor, CROs have inspired a generation of ‘green’ small-molecule oxidation catalysts, the utility of which is the chemoselective oxidation of alcohols using only aerobic oxygen as a cosubstrate. In addition, the capacity of these CROs to generate hydrogen peroxide is of increasing biological interest in the context of recalcitrant plant cell wall degradation by fungal saprotrophs and phytopathogens [8] , [9] . Specifically, peroxide production is believed to be coupled to lignolytic peroxidases as well as non-enzymatic Fenton chemistry [8] . To catalyse the oxidation of their eponymous substrates with concomitant hydrogen peroxide production, glyoxal oxidases and galactose 6-oxidases have a conserved mononuclear copper-radical active site comprising a crosslinked cysteine–tyrosine residue together with one unmodified axial tyrosine side chain and two histidine side chains as additional coordinating residues [8] , [10] . In galactose 6-oxidase, experimental evidence suggests that the first half-reaction involves proton transfer from O-6 of galactose to the axial tyrosine anion, hydrogen atom transfer (HAT) from C-6 of galactose to the tyrosine–cysteine radical cofactor and electron transfer from the carbohydrate to generate the aldehyde and Cu(I). To complete the catalytic cycle, the second half-reaction is proposed to involve inner-sphere electron transfer from Cu(I) to oxygen to yield superoxide, HAT from the phenolic hydroxyl group of the Tyr–Cys cofactor to the superoxide to produce metal-bound hydroperoxide and proton transfer from the axial tyrosine to hydroperoxide to produce hydrogen peroxide and the re-oxidized, active Cu(II)-radical state of the enzyme ( Fig. 1 ) [11] . These observations are reflected in the known detailed mechanisms of a range of bio-inspired small-molecule copper complexes that act as catalysts for the aerobic oxidation of alcohols [12] . In contrast to galactose 6-oxidase, the mechanism of aldehyde oxidation by glyoxal oxidase has not been studied in as great detail; however, it has been suggested that this enzyme may in fact react with the hydrated, gem -diol form of the substrate via an analogous mechanism [13] , [14] . 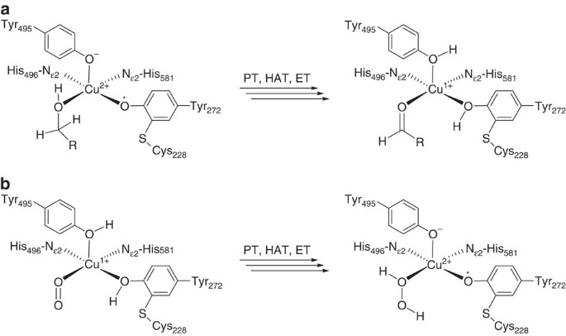Figure 1: Abbreviated mechanism of galactose oxidase. (a) The first half-reaction in which the enzyme is reduced while oxidizing the alcohol to the aldehyde. (b) The second half-reaction reduces O2to H2O2while oxidizing copper1+to the resting +2 oxidative state (reviewed in ref.10; see ref.11for a detailed mechanism). ET, electron transfer; PT, proton transfer. Figure 1: Abbreviated mechanism of galactose oxidase. ( a ) The first half-reaction in which the enzyme is reduced while oxidizing the alcohol to the aldehyde. ( b ) The second half-reaction reduces O 2 to H 2 O 2 while oxidizing copper 1+ to the resting +2 oxidative state (reviewed in ref. 10 ; see ref. 11 for a detailed mechanism). ET, electron transfer; PT, proton transfer. Full size image As a complement to the activity-based Enzyme Commission classification, the sequence-based Carbohydrate-Active Enzymes (CAZy; www.cazy.org ) classification has, since its inception in 1991, significantly augmented the mapping of structure–function relationships among enzymes involved in glycosidic bond formation and cleavage [15] . More recently, the CAZy classification has been extended to encompass a range of Auxiliary Activity (AA) families (currently 13), which comprise a diversity of redox enzymes acting on polyphenolics and carbohydrates [16] . Among these families, Auxiliary Activity Family 5 (AA5) encompasses known (methyl)glyoxal oxidases in subfamily 1 (AA5_1) and galactose 6-oxidases in subfamily 2 (AA5_2) [16] ( Fig. 2 ). The occurrence of AA5 family enzymes is wide: as of October 2015, AA5 members in the public CAZy database comprised ∼ 90 fungal sequences in subfamilies 1 and 2, as well as a large number of bacterial AA5_2 members ( ca. 270) primarily from Burkholderia sp. genome-sequencing efforts (see http://www.cazy.org/AA5_subfamilies.html , ref. 16 ). 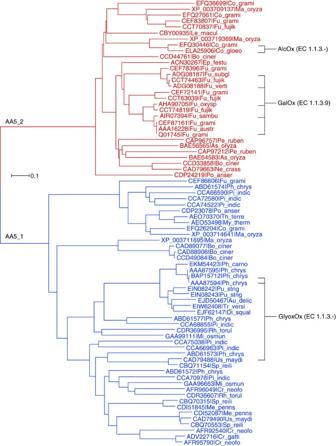Figure 2: Phylogeny of AA5. Subfamilies 1 (AA5_1) and 2 (AA5_2) are indicated. GenBank identifiers (UniProt identifier Q01745 in the case of theF. graminariumGalOx) are given for all sequences available in the public release of the CAZy Database16as of June 2015; full genus and species names of source organisms can be obtained from the respective GenBank entries. AA5 members for which enzymological data have been conclusively linked to protein sequence are indicated as (methyl)glyoxal oxidases (GlyoxOx)9,13,14,17,18, galactose oxidases (GalOx; refs19,27,34,35,68and references therein), or general alcohol oxidases (AlcOx; this study). Figure 2: Phylogeny of AA5. Subfamilies 1 (AA5_1) and 2 (AA5_2) are indicated. GenBank identifiers (UniProt identifier Q01745 in the case of the F. graminarium GalOx) are given for all sequences available in the public release of the CAZy Database [16] as of June 2015; full genus and species names of source organisms can be obtained from the respective GenBank entries. AA5 members for which enzymological data have been conclusively linked to protein sequence are indicated as (methyl)glyoxal oxidases (GlyoxOx) [9] , [13] , [14] , [17] , [18] , galactose oxidases (GalOx; refs 19 , 27 , 34 , 35 , 68 and references therein), or general alcohol oxidases (AlcOx; this study). Full size image Strikingly, the recent CAZy classification of AA5 reveals a paucity of sequence-correlated functional and structural information in this family. Indeed, since the initial discovery nearly 30 years ago of (methyl)glyoxal oxidase activity in the white-rot basidiomycete Phanerochaete chrysosporium [8] , only the archetype Pch Glx1 (refs 13 , 14 , 17 ), a strain-specific point variant [18] , and a homologue from the phytopathogenic fungus Ustilago maydis [9] have been recombinantly produced and enzymatically characterized, while no three-dimensional (3D) structures have been solved for any AA5_1 members [8] . Studies on AA5_2 members have essentially exclusively focused on the archetypal galactose 6-oxidase from the cereal head blight ascomycete Fusarium graminearum (anamorph of Gibberella zeae ), encompassing recombinant production, biochemical and kinetic analyses, spectroscopy, crystallography, enzyme engineering and applications [5] , [10] . Recently, four additional AA5_2 members from other Fusarium species have been biochemically defined as galactose 6-oxidases (ref. 19 and references therein), yet the number and phylogenetic diversity of characterized AA5 members remain low ( Fig. 2 ). Intriguingly, the 3D structure of a Streptomyces lividans AA5 member (not associated with either subfamily) involved in hyphal morphogenesis, but of unclear substrate specificity, was very recently described [20] . However, the diversity and evolution of substrate specificity in AA5 is largely uncharted [8] , thereby limiting enzyme discovery for biotechnological applications [1] , [6] . Accordingly, a key question arises over whether the scope of activity has yet been fully defined for AA5 enzymes. This notion is given further weight from a small handful of early studies of AA5 enzymes, which hint at a limited number of aliphatic alkyl alcohols being substrates for AA5 enzymes, albeit at extremely low levels of activity [21] , [22] , [23] . There are also several studies that show that activated alcohols, such as benzyl and allylic alcohols, are oxidized by these enzymes to yield conjugated aldehyde products [10] . Other work has demonstrated that AA5 mutants are active catalysts for the aerobic oxidation of both activated and unactivated secondary alcohols [24] , [25] . These studies are in addition to early work on the wide range of galactosides that act as substrates [26] , [27] . The most compelling signal, however, comes from chemical studies of the suite of small-molecule catalysts that incorporate the unique active site features of AA5 family enzymes, most notably the presence of a copper-coordinating redox-active ligand [12] . Several of these catalysts are capable of oxidizing unactivated aliphatic alcohols at high rates, thus indicating that wild-type AA5 members may also catalyse the oxidation of a range of alcohol substrates, which—if true—expands the biochemical role of AA5 enzymes and their potential biotechnological applications. Originally motivated, therefore, by an interest to discover new galactose 6-oxidases with improved recombinant production, biochemical and kinetic properties for polysaccharide modification [28] , [29] , [30] , we selected two homologous gene products from the recently sequenced plant pathogens Colletotrichum graminicola M1.001 (refs 31 , 32 ) and C. gloeosporioides Nara gc5 (ref. 33 ) for functional characterization (see also http://www.colletotrichum.org/genomics/ ). This choice was driven, in part, by the smaller size and novel predicted domain structure of these proteins—both enzymes lack the N-terminal family 32 Carbohydrate-Binding Module (CBM32) found in the F. graminearum GalOx ( Fgr GalOx)—as well as their apparent phylogenetic distance from the Fgr GalOx in a separate clade of AA5_2. As described hereafter, our studies demonstrate that both copper-dependent enzymes had extremely feeble activity on galactose and galactosides, but instead oxidize a range of primary alkyl alcohols (activated and unactivated) with concomitant generation of H 2 O 2 . Crystallography of the C. graminicola AlcOx as the second unique structural representative of AA5 revealed a conserved overall fold and active site vis-à-vis the archetypal Fgr GalOx catalytic module, while detailed comparative structural and phylogenetic analyses revealed the key features in the evolution of AA5 enzymes. These findings now extend the biochemical and structural coverage of AA5, highlight a greater catalytic diversity of AA5_2 members than had been previously appreciated and deliver new biocatalysts for potential applications in alcohol oxidation under mild aqueous conditions without the need for nucleotide cofactors and basic activators. Phylogenetic relationships of Cgr AlcOx and Cgl AlcOx in AA5 Sequence alignment of 75 AA5 members in isolation from all predicted signal peptides and other ancillary protein modules, constituting the complete cohort of fungal sequences in the public CAZy Database, resulted in phylogenetic tree revealing a clear distinction between AA5 Subfamily 1 (AA5_1) and Subfamily 2 (AA5_2; Fig. 2a , see also http://www.cazy.org/AA5_subfamilies.html ). Mapping enzyme activity data on this phylogeny reveals that the three (methyl)glyoxal oxidases fall into AA5_1 and the five Fusarium spp. galactose 6-oxidases fall into a clade of AA5_2. In addition, within AA5_2, the gene products of C. graminicola M1.001 locus GLRG_05590.1 (UniProt E3QHV8; GenBank EFQ30446; hereafter ‘ Cgr AlcOx’) and C. gloeosporioides Nara gc5 locus CGGC5_13025 (GenBank ELA25906; hereafter ‘ Cgl AlcOx’) were selected for enzyme characterization due to significant amino-acid sequence differences with the archetypal galactose 6-oxidase from F. graminearum , Fgr GalOx (Genbank AAA16228.1), including the absence of the N-terminal CBM32 of Fgr GalOx. Amino-acid sequence alignment reveals that Cgr AlcOx and Cgl AlcOx share 82% sequence identity with each other, but only 46% and 48% identity, respectively, to the AA5 module of GalOx from F. graminearum ( Supplementary Fig. 1 ). All AA5 sequences known to date contain the key active-site residues of Fgr GalOx, namely, C228 and Y272 that combine to form the unique crosslinked thioether-tyrosyl cofactor, and Y495, H496 and H581 that also coordinate to the copper ion [34] (see also Fig. 1 and Supplementary Fig. 1 ). Production of Cgr AlcOx and Cgl AlcOx by Pichia pastoris The methylotrophic yeast P. pastoris was chosen as the recombinant production host for both AA5 members, based on previous work with Fgr GalOx (refs 28 , 29 ). During cloning, predicted native secretion signal peptides were replaced with the Saccharomyces cerevisiae α-factor secretion signal for extracellular secretion; hereafter, all residue numbering refers to that of the predicted mature sequence of the native protein shown in Supplementary Fig. 1 . Maximum production (30–40 mg l −1 with specific activities towards 1-butanol of 71 and 55 U mg −1 for Cgr AlcOx and Cgl AlcOx, respectively) was generally observed after 3 days with induction using 1% methanol in BMMY media at 16 °C in well-aerated, baffled shake flasks. As previously observed for Fgr GalOx production [29] , the addition of copper (II) sulfate was essential to obtain maximal activity, with 0.05, 0.2 and 0.5 mM CuSO 4 all providing similar benefit, whereas 2 mM CuSO 4 was detrimental to production (data not shown); 0.05 mM CuSO 4 was used routinely. Subsequent two-step purification by immobilized metal-ion affinity and size exclusion chromatographies yielded 35 mg ml −1 of Cgr AlcOx and 14 mg ml −1 of Cgl AlcOx with specific activities of 119 and 86 U mg −1 , respectively, towards the standard substrate 1-butanol. These enzyme preparations were found to be >90% pure using SDS–PAGE, and enzymatic deglycosylation indicated that both enzymes were N-glycosylated ( Supplementary Fig. 2 ). The observation of recombinant protein glycosylation by the yeast host is consistent with analysis by the NetNGlyc server (ver. 1.0), which predicted two glycosylation sites in Cgr AlcOx (N58 and N186) and Cgl AlcOx (N58 and N191). After purification and treatment with EDTA, residual tightly bound copper was present in the as-purified proteins, which could be detected using electron paramagnetic resonance (EPR) spectroscopy ( vide infra ) and quantified using EPR spin quantitation to be 0.9±0.1 equivalents of Cu(II) per monomer. Cgr AlcOx and Cgl AlcOx are competent alcohol oxidases On the basis of the common membership of Cgr AlcOx and Cgl AlcOx in the same subfamily as Fgr GalOx, we anticipated that these enzymes would likewise catalyse the oxidation of the primary alcohol in galactose and galactosides to the corresponding aldehyde. Initial activity screening of Cgr AlcOx against a panel of carbohydrate substrates reveals an extremely weak activity towards galactose, raffinose and xyloglucan (<0.3 U mg −1 ), which are good substrates for Fgr GalOx (refs 27 , 29 ). Lactose, glucose, xylose and arabinose are similarly poor substrates, yet glycerol was oxidized with a 50-fold greater specific activity than galactose ( Fig. 3 ). This discovery prompted us to test the activity against a wider selection of alcohols ( Table 1 ), which reveal a significantly greater (150-fold) specificity, based on k cat / K m values, of Cgr AlcOx for aliphatic primary alcohols such as 1-butanol compared with polyols such as glycerol, xylitol and sorbitol. A similar trend is observed for the homologous Cgl AlcOx ( Table 1 ). Indeed, plots of initial rate kinetics versus substrate concentration are classically Michaelian for all competent substrates, except for those with apparently high K m values, which appear as strictly linear plots (representative data for Cgr AlcOx are shown in Supplementary Fig. 3 ; similar data for Cgl AlcOx are not shown). 1-Butanol was selected as the benchmark substrate and was used to determine the pH-rate profile and temperature stability of Cgr AlcOx and Cgl AlcOx. Both enzymes exhibit bell-shaped pH-rate profiles, consistent with two ionizable groups involved in catalysis as proposed for Fgr GalOx (ref. 11 ), with basic pH optima ( Supplementary Fig. 4 ). Both enzymes are significantly stable below 30 °C, but rapidly lose activity above 50 °C, in keeping with the mesophilic nature of their natural host ( Supplementary Fig. 5 ). A pH of 8.0 and temperature of 23 °C were used for all subsequent enzymology, including the generation of all data in Table 1 . 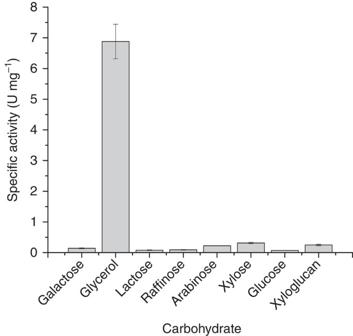Figure 3: Initial activity screen ofCgrAlcOx against carbohydrates. Saccharides and glycerol were assayed at 50 mM and xyloglucan was assayed at 1 g l−1. Results shown are averages of duplicate measurements from a single experimental replicate; error bars represent s.d.’s. Figure 3: Initial activity screen of Cgr AlcOx against carbohydrates. Saccharides and glycerol were assayed at 50 mM and xyloglucan was assayed at 1 g l −1 . Results shown are averages of duplicate measurements from a single experimental replicate; error bars represent s.d.’s. Full size image Table 1 Substrate specificity* of Cgr AlcOx and Cgl AlcOx. Full size table The extensive panel of kinetic data for Cgr AlcOx in Table 1 reveals general substrate preferences with respect to the benchmark 1-butanol, which are mirrored in the homologue Cgl AlcOx. Extension of the alkyl chain to pentyl, hexyl or heptyl has a limited effect on k cat values and only slightly reduces K m values (less than fourfold across the series) with correspondingly little effect on k cat / K m values. On the other hand, systematic reduction in alkyl chain length from butyl to methyl greatly increases K m values and reduces k cat / K m values, with methanol being a poor substrate ( k cat / K m is 700-fold lower than that for 1-butanol). It is interesting to note here that activity of the AA5 AlcOx enzymes on methanol does not significantly complicate protein production under control of the methanol-dependent AOX promoter in P. pastoris under shake flask conditions. However, high-yield production using a continuous methanol feed in a fermenter was unsuccessful for Cgr AlcOx (data not shown). Product analysis clearly indicated that 1-butanol is oxidized to butanal by Cgr AlcOx ( Supplementary Fig. 6 ); however, we were routinely unable to obtain substrate conversions beyond 30%. This was despite several attempts including the use of high enzyme loadings and the addition of a large excess of catalase to breakdown the peroxide co-product; the presence of horseradish peroxidase (HRP, previously shown to aid Fgr GalOx substrate conversion [30] ) also has no effect (data not shown). The reason for this is unclear in light of the complete conversion of conjugated primary alcohols ( vide infra ). In contrast to primary alkanols, AA5 AlcOx oxidation of the secondary alkanols 2-butanol and 2-propanol is extremely poor. Substrate saturation could not be obtained and k cat / K m values extracted from linear plots of v o versus [S] are at least 3,500-fold lower than that for 1-butanol ( Table 1 ). On the other hand, 1,3-propanediol and 1,4-butanediol are competent substrates, the kinetics of oxidation of which are almost identical to the corresponding 1-alkanols. 1,2-propanol and the linear polyols glycerol, xylitol and sorbitol are comparatively poor substrates, indicating that, while 1,3-diol substitution is well tolerated by these AA5 AlcOxs, 1,2-diol substitution is not. Notably, in all cases, 1,2-diol substrates have nearly identical k cat values to 1-butanol and the other diols; however, K m values are substantially increased, yielding up to 300-fold lower specificity constants ( k cat / K m values, Table 1 ). Product analysis using glycerol as a substrate for Cgr AlcOx again reveals oxidation of the primary alcohol, as observed for 1-butanol, yielding glyceraldehyde hydrate in this case ( Supplementary Fig. 7 ). As with 1-butanol, we again were unable to effect complete conversion of the substrate despite repeated attempts, including optimization of reaction conditions. The detrimental effect of 2-substitution is mirrored in the kinetics of (±)-2-methyl-1-butanol and (S)-(-)2-methyl-1-butanol which, despite exhibiting similar k cat values to 1-butanol, has 20- and 125-fold higher K m values and correspondingly poorer k cat / K m values, respectively ( Table 1 ). Product analysis using NMR indicates that (±)-2-methyl-1-butanol is converted to the corresponding aldehyde ( Supplementary Fig. 8 ), yet, as for 1-butanol and glyceraldehyde, conversion levels >30% could not be obtained. The observed sixfold difference in k cat / K m values suggests enantioselectivity for (R)-2-methyl-1-butanol (commercially unavailable), which is also indicated by chiral GC/MS analysis of the products; yet, the low substrate conversion prevents quantitative determination of an enantiomeric-excess value. The hydroxy-amino-acid serine is not detectibly oxidized by either AlcOx, and the buffer TRIS is only weakly oxidized by Cgr AlcOx ( Table 1 ). Benzyl alcohol is an excellent substrate for both AA5 AlcOx enzymes, exhibiting kinetic constants similar to 1-butanol ( Table 1 ). In contrast to the 1-alkanols, oxidation of benzyl alcohol to benzaldehyde by Cgr AlcOx is essentially complete ( Supplementary Fig. 9 ). Moreover, 4-hydroxylation, 4-methoxylation and 2,3-dimethoxylation of the aromatic ring abolishes activity below the limit of detection of the assay at high enzyme loadings (200 ng). 2-phenyl-ethan-1-ol is a competent substrate, with kinetic constants comparable to those of 1-propanol. Like benzyl alcohol, cinnamyl alcohol is an excellent substrate for both AA5 AlcOx enzymes, with Cgr AlcOx demonstrating an especially low K m value ( Table 1 ). NMR analysis indicates the facile (>99%) conversion of cinnamyl alcohol by Cgr AlcOx to cinnamaldehyde ( Supplementary Fig. 10 ), which was also apparent because of the fragrance of the product. Again, in analogy with benzyl alcohol, hydroxylation and methoxylation of the aromatic ring are not tolerated, such that the monolignols p -coumaryl alcohol, sinapyl alcohol and coniferyl alcohol are all not detectibly oxidized by the either AA5 AlcOx at high enzyme loadings. The oxidation of hexa-2,4-diene-1-ol by both Cgr AlcOx and Cgl AlcOx exhibits excellent kinetics, including the highest k cat value of all substrates tested and a low K m value (essentially identical to cinnamyl alcohol, Table 1 ), as well as near-complete substrate conversion ( Supplementary Fig. 11 ). Notably, the k cat / K m value of Cgr AlcOx for hexa-2,4-diene-1-ol is 4.7-fold higher than that for the corresponding 1-hexanol and over an order of magnitude higher than that for 1-butanol. The hydroxylated terpene geraniol, which contains a 3-methyl substituent on the double bond, is also a good substrate for Cgr AlcOx, with a k cat / K m value similar to those of the 1-alkanols with C 4 chains and higher. Removal of potential conjugation in the product, in the case of cis-3-hexen-1-ol, results in a substrate specificity of Cgr AlcOx again similar to the 1-alkanols. Tertiary structure of Cgr AlcOx and metal site geometry The 3D structure of Cgr AlcOx was solved using the homologous two domains of Fgr GalOx as the model. Surprisingly, given the difficulty of demetallating with EDTA, crystals grown in 0.1 M imidazole were copper-free. A copper-containing structure was eventually obtained from different conditions augmented with a 15-day soak with powdered CuSO 4 in the droplets. The apo and Cu structures have an r.m.s.d of 0.3 Å (and all subsequent discussions use the Cu crystal structure as a reference). As expected, the Cgr AlcOx structure displays two domains composed mainly of β-sheets and connecting loops ( Fig. 4a,b ). The N terminus (residues 1–370) displays seven ‘Kelch’ motifs, which together form a classical seven-bladed β-propeller (and which contains the active centre, vide infra ). The C-terminal domain, comprising residues 371–488, forms an immunoglobulin-like beta sandwich domain from which residues 418–430 pierce the N-terminus propeller axis as a finger, providing the apical His423 that is one of the copper coordination residues (described below). As expected for proteins with ∼ 40–50% sequence identity, the two common domains of Cgr AlcOx and Fgr GalOx are extremely similar with an r.m.s.d of 0.98 Å over 465 equivalent Cα atoms (48% identical amino acids); the best match was with the Fgr GalOx W290F variant (PDB code 2EIC (ref. 35 ), PDBeFOLD Q score 0.64). The most obvious structural difference between Fgr GalOx and Cgr AlcOx is that the latter lacks the N-terminal CBM32 (ref. 34 ; Fig. 4c ). In other enzymes, CBM32 members are generally known to bind galactosyl residues [36] , and indeed galactose binding was revealed in the seminal crystal structure of Fgr GalOx (ref. 34 ). In light of the kinetic data, the absence of this module in both Cgr AlcOx and Cgl AlcOx is entirely consistent with the observed non-carbohydrate substrate specificity of these enzymes. 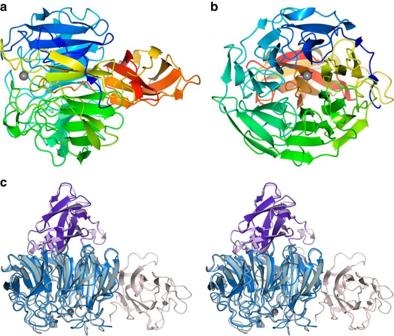Figure 4: 3D structure ofCgrAlcOx. (a) At the N terminus (colour-ramped blue to yellow), seven Kelch motifs enclose the copper-binding site in a β-propeller arrangement, while the C terminus displays a nine-stranded β-barrel (orange to red). (b) Orthogonal view. The Cu ion is showed as a grey-shaded sphere. (c) Overlap ofCgrAlcOx (dark) andFgrGalOx (pale, 2EIE), in divergent (‘wall-eyed’) stereo highlighting the additional N-terminal CBM32 domain of the latter (pale pink). Figure 4: 3D structure of Cgr AlcOx. ( a ) At the N terminus (colour-ramped blue to yellow), seven Kelch motifs enclose the copper-binding site in a β-propeller arrangement, while the C terminus displays a nine-stranded β-barrel (orange to red). ( b ) Orthogonal view. The Cu ion is showed as a grey-shaded sphere. ( c ) Overlap of Cgr AlcOx (dark) and Fgr GalOx (pale, 2EIE), in divergent (‘wall-eyed’) stereo highlighting the additional N-terminal CBM32 domain of the latter (pale pink). Full size image Consistent with the EPR quantitation of 0.9±0.1 equivalents of Cu(II) per protein, the crystal structures of copper-containing Cgr AlcOx and Cgl AlcOx show the presence of one mononuclear copper site. The copper coordination site of Cgr AlcOx is essentially as described for Fgr GalOx. Copper coordination is provided by Tyr120, Tyr334, His335 and His423 at the centre of the β-propeller ( Fig. 5a ). As found in the homologous galactose 6-oxidase, Cys73 is linked to Tyr120 (equating to Cys228 and Tyr272 in Fgr GalOx) via a thioether bond. The observed ligation geometry of the copper site is three coordinate and T-shaped, with short interactions with Tyr120 (Cu-O 2.1 Å), His423 (Cu-N 2.2 Å) and His335 (Cu-N 2.4 Å), while a fourth interaction with Tyr334 (Cu-O 2.8 Å) is too long to be considered a bonding interaction. 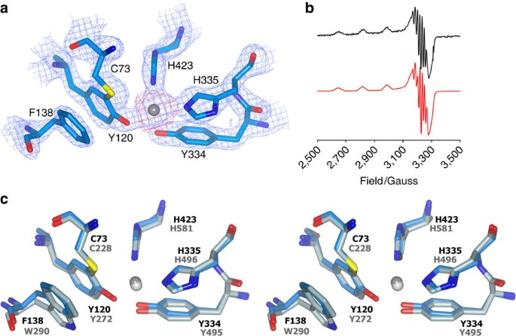Figure 5: Active site ofCgrAlcOx. (a) Observed electron density map for the active site, maximum likelihood (REFMAC) weighted 2Fobs–Fcalcmap contoured at 0.59 Å3Da−1, with the anomalous difference density map (red,λ=0.979 Å) contoured at 2σ. Copper is coordinated by residues Y120, Y334, H335 and H423 in the centre of the N-terminal β-propeller. (b) X-band EPR spectrum (9.3 GHz, 155 K) of Cu-CgrAlcOx in 10% v/v glycerol (black) with simulation (red). The spectrum ofCglAlcOx was identical (Supplementary Fig. 12). (c) Divergent stereoscopic view of the overlay ofCgrAlcOx (dark) andFgrGalOx (pale) copper-binding centres. F138 inCgrAlcOx is substituted by W290 inFgrGalOx. Figure 5: Active site of Cgr AlcOx. ( a ) Observed electron density map for the active site, maximum likelihood (REFMAC) weighted 2 F obs – F calc map contoured at 0.59 Å 3 Da −1 , with the anomalous difference density map (red, λ =0.979 Å) contoured at 2 σ . Copper is coordinated by residues Y120, Y334, H335 and H423 in the centre of the N-terminal β-propeller. ( b ) X-band EPR spectrum (9.3 GHz, 155 K) of Cu- Cgr AlcOx in 10% v/v glycerol (black) with simulation (red). The spectrum of Cgl AlcOx was identical ( Supplementary Fig. 12 ). ( c ) Divergent stereoscopic view of the overlay of Cgr AlcOx (dark) and Fgr GalOx (pale) copper-binding centres. F138 in Cgr AlcOx is substituted by W290 in Fgr GalOx. Full size image EPR analysis was performed on as-isolated Cgr AlcOx and Cgl AlcOx to determine the electronic structure of the resting oxidized state. Both proteins gave identical spectra ( Supplementary Fig. 12 ). These show, in accord with previous EPR studies on galactose 6-oxidase enzymes [35] , [37] , [38] , that the SOMO of the resting state is largely d( x 2 – y 2 ) in character, indicating a single copper site with an axial coordination geometry ( g z ≠ g x = g y ; Fig. 5b ). Unusually, there is a clear resolution of super-hyperfine coupling to the coordinating nitrogen atoms, revealing a well-ordered active site with some covalence in the Cu-N bonds. The spectrum could be satisfactorily simulated using a CuN 2 spin system with g z =2.29 and |A z |=178 × 10 −4 cm −1 and g x = g y =2.06, |A x |=38 × 10 −4 cm −1 , |A y |=13 × 10 −4 cm −1 , placing the copper site squarely within the Type 2 definition of Peisach and Blumberg [39] . Second differential plots afforded accurate values of the super-hyperfine coupling constants to the coordinating nitrogen atoms of 14 × 10 −4 cm −1 , in accord with the expected values for coupling to two sp 2 -hybridized nitrogen atoms [40] . Previous studies on an inactive, oxidized state of Fgr GalOx, which contains a Cu(II) site and a 1-electron reduced (that is, neutral) Cys-Tyr cofactor, produced a low-temperature EPR spectrum very similar to that observed for as-isolated Cgr AlcOx and Cgl AlcOx ( g z =2.29 and A z =191 × 10 −4 cm −1 ) including well-defined Cu-N coupling [35] , [37] , [41] , [42] . Thus, we conclude that as-isolated Cgr AlcOx and Cgl AlcOx also contain a Cu(II) site and a one-electron reduced form of the Cys-Tyr cofactor, and the active site structure observed using X-ray crystallography likely reflects this inactive state. As has been demonstrated for Fgr GalOx, this inactive state can be activated under typical assay conditions. We investigated the redox properties of the inactive resting state of Cgr AlcOx by incubating the enzyme with the reductant sodium dithionite and the oxidant potassium ferricyanide ( Supplementary Fig. 13 ). On addition of dithionite ( E o =−660 mV) [43] to resting Cgr AlcOx, a loss of ∼ 70% of the EPR spin intensity is observed, accompanied by a colour change from blue to colourless, showing that dithionite reduces the resting inactive state. However, Cgr AlcOx is not oxidized by ferricyanide ( E o =+436 mV) [44] , which contrasts previous observations on Fgr GalOx (ref. 37 ). This difference indicates a lower potential of the Cys-Tyr cofactor in Cgr AlcOx compared with the archetypal GalOx, which may account for the ability of the AlcOx enzymes to oxidize unactivated alcohol substrates. The structural origin of the lower redox potential of the Cys-Tyr cofactor in Cgr AlcOx is discussed below. The main difference between the Cgr AlcOx and Fgr GalOx active sites is that a key tryptophan (Trp290) in Fgr GalOx is replaced by a phenylalanine (Phe138) in Cgr AlcOx ( Fig. 5c , cf. Supplementary Fig. 1 ). Previous studies of the activity of Trp290 mutants of Fgr GalOx have indicated a dramatic loss of oxidative capacity on mutation, which is correlated to significantly higher K m values for the natural substrate galactose with the Fgr GalOx W290G/F mutants ( ∼ 200–300 mM compared with 82 mM for wild type), presumably because of the loss of a hydrogen-bonding interaction between W290 and a remote hydroxyl group of the substrate [35] . The natural occurrence of Phe in Cgr AlcOx and Cgl AlcOx may help account for the very low activity of these enzymes on carbohydrate substrates. The observed K m values of 0.2–10 mM for Cgr AlcOx with aliphatic alcohols provide an indication that a lack of hydrogen-bonding capacity in residue 290 does not compromise binding of aliphatic substrates (assuming K m reflects K s ). In addition, Trp290 in Fgr GalOx has been implicated in stabilizing the radical form of the Cys-Tyr cofactor, although substitution with either Phe (the wild-type residue in Cgr AlcOx) or Gly also stabilized the tyrosine radical with retention of catalytic activity, while other substitutions were detrimental to the enzyme [35] . A decrease in the stability of the oxidized radical cofactor in Cgr AlcOx compared with Fgr GalOx, because of poorer stabilization by Phe compared with Trp, would account for the lower redox potential of the inactive state of Cgr AlcOx ( vide supra ). This also is consistent with small-molecule studies, which suggest that aromatic stacking interactions may tune the redox potential of radicals. Thus, substitution of Trp290 by Phe may enhance the ability of the enzyme to oxidize unactivated alcohols by enhancing the ability of the Cys-Tyr cofactor to accept a hydrogen atom during the HAT step [45] , [46] . Indeed, the apparent second-order rate constants for the oxidation of longer-chain primary aliphatic alcohols by Cgr AlcOx and Cgl AlcOx are of the order of 10 4 –10 5 M −1 s −1 , some 10–100 times higher than that for oxidation of galactose by Fgr GalOx, suggesting that the active site in these enzymes is tuned for better reactivity with aliphatic substrates. In the other direction, production of the Cgr AlcOx F138W variant causes an essentially complete loss of the ability to oxidize alkanols, while the ability to oxidize substrates with extended conjugation (2,4-hexadienol and cinnamyl alcohol) increases ca. 1.2-fold. At the same time, activity towards benzyl alcohol is reduced ca. twofold ( Supplementary Fig. 15b ). The precise reason for this altered specificity is unclear, and indeed the opposite mutation in Fgr GalOx (W290F) has been also shown to reduce turnover and increase the Michaelis constant for the primary substrate, galactose, as discussed above [35] . Overall, it is clear that this second-shell coordination residue plays a central role in substrate recognition and catalysis through the presence or absence of a hydrogen bond to the substrate and through a stacking interaction with the Cys-Tyr cofactor ( Fig. 4 ), yet it is not primarily responsible for modulating between galactose 6-oxidase and general alcohol oxidase activity in AA5_2. More distant from the active centre, four loop regions show significant differences in position between Fgr GalOx and the AlcOx enzymes ( Supplementary Fig. 14 ). Three of these are close to the copper site and were selected for chimeric loop substitutions. To explore the effect of these differences on substrate specificity in AA5_2, these elements were introduced individually on the Cgr AlcOx scaffold. Unfortunately, none of the four new variants exhibits a gain of GalOx activity, although these mutations strongly affect the substrate specificity of Cgr AlcOx, as judged by screening specific activity at near-saturating substrate concentrations on a selection of alcohols ( Supplementary Fig. 15 ). Of the three active-site loop variants, the replacement of Loop 3 in Cgr AlcOx with that of Fgr GalOx has remarkably little effect on catalysis, with specific activity values for all substrate tested reduced approximately equally to 50–75% of wild-type levels. Loop 1 and Loop 2 variants, on the other hand, are significantly impaired with activities on all substrates tested reduced to ca. 10 and ca. 1% of wild-type levels, respectively ( Supplementary Fig. 15c–e ). Although all loop variant proteins appear to be well behaved following purification, including with regard to solubility, we are unable to rule out folding problems leading to a fraction of inactive protein as one source of the observed reductions in specific activities. Nonetheless, as for the Cgr AlcOx F138W variant, it is clear that none of these loops is individually responsible for the chemoselectivity of AA5_2 members. Resolving protein structure–function relationships in AA5_2 will therefore require far more extensive mutagenesis efforts, including the production of combinations of variants. Many Colletotrichum species are hemibiotrophs that cause anthracnose diseases in a wide range of plant hosts, including many important food crops. For example, anthracnose leaf blight and stalk rot of maize caused by C. graminicola have been estimated to result in annual yield losses of ca. 6% in the United States alone [31] . Consequently, there has been recent, sustained interest in Colletotrichum genomics to understand the unique biology of specific host–pathogen interactions (refs 31 , 32 , 47 and references therein). In the present work, we have utilized this wealth of sequence data and precedence from small-molecule copper-containing oxidation catalysts to discover two novel alcohol oxidases from CAZy AA5, which provides essential biochemical data to seed bioinformatics analyses, understand host biology and expand the range of biocatalysis for applications. Indeed, the classification of Cgr AlcOx and Cgl AlcOx in the same subfamily as Fgr GalOx may result in the erroneous extrapolation of functional annotation as galactose 6-oxidases to these enzymes. For example, Cgl AlcOx is currently listed under the NCBI GenBank ID ELA25906.1 as a ‘galactose oxidase precursor.’ Although our enzymological data clearly demonstrate that Cgr AlcOx and Cgl AlcOx are not galactose 6-oxidases, they do share a common Kelch-repeat β-propeller fold, conserved copper and crosslinked Cys-Tyr cofactor active site and mechanistic commonality with their closest AA5_2 relative, the archetypal Fgr GalOx. Caution is therefore warranted in the annotation of enzyme function on the basis of primary and tertiary structural data alone. Cgr AlcOx and Cgl AlcOx exhibit a broad substrate range, resulting in the oxidation of saturated and unsaturated primary alcohols to the corresponding aldehydes with the concomitant production of hydrogen peroxide from molecular oxygen. Comparison with several mechanistically diverse alcohol oxidases characterized on the same substrates reveals that Cgr AlcOx and Cgl AlcOx are competent enzymes. For example, the second-order rate constants ( k cat / K m ) of the oxidation of benzyl alcohol, cinnamyl alcohol and 2,4-hexadiene-1-ol by both enzymes are equivalent to or significantly greater than the FAD-dependent aryl-alcohol oxidase from Pleurotus eryngii [48] ( Supplementary Table 2 ). Benzyl alcohol is also known to be a substrate for Fgr GalOx (ref. 49 ); however, Cgr AlcOx and Cgl AlcOx demonstrate 330- and 195-fold higher k cat / K m values, respectively, for this aryl alcohol. Cgr AlcOx has a k cat / K m value for the oxidation of 1-heptanol that is a notable three orders of magnitude higher than for the FAD-dependent AOX from Aspergillus terreus [50] , while both Cgr AlcOx and Cgl AlcOx are much less efficient at methanol oxidation than an FAD-dependent Gloeophyllum trabeum AOX [51] ( Supplementary Table 2 ). Although the natural alcohol substrate is currently unresolved (for example, long-chain alcohols representing cuticle waxes were too insoluble to be tested), we speculate that these enzymes may function in the context of the plant cell wall by generating highly diffusible reactive oxygen species for polysaccharide and lignin oxidation (especially in combination with Fenton chemistry), as has been proposed for glyoxal oxidase and other AOXs [8] , [51] . In sum, the kinetic data reveal a pattern of reactivity of alcohols with either Cgr AlcOx or Cgl AlcOx in which unactivated aliphatic alkyl alcohols become better substrates with increasing chain length. Activated alcohols, such as benzyl and hexa-2,4-diene-1-ol, are excellent substrates, although they do not exhibit significantly higher k cat values compared with unactivated alcohols. As such, further in-depth mechanistic and kinetic studies are required to elucidate the detailed mechanistic pathway of Cgr AlcOx and Cgl AlcOx. While Cgr AlcOx and Cgl AlcOx are unlikely to exhibit a vastly different overall mechanism, the observation that unactivated alkyl alcohols are uniquely competent substrates for the AlcOx enzymes vis-à-vis the archetypal Fgr GalOx (ref. 23 ) raises the possibility that the key step, canonically thought to involve HAT by a coordinated Cys-Tyr radical cofactor, may differ among AA5 members. Intriguingly, studies of small-molecule copper catalysts for the aerobic oxidation of alcohols indicate that complexes that perform this oxidative step with a coordinated Tyr radical do not oxidize unactivated alcohols. At the same time, other oxidative mechanisms are known, including direct reaction of a copper-bound oxygen species with the alcohol, or the oxidation of unactivated alcohols by copper-TEMPO catalysts in which HAT is affected by a reactive radical species not directly coordinated to the copper [12] . These observations regarding the reactivity of small-molecule catalysts raise the possibility that the relative stability and positioning of the Cys-Tyr cofactor in the active site may be a key factor in tuning reactivity and modulating the potential range of α-C–H bonds in primary alcohols that can be cleaved by AA5 members, a point previously noted in studies of Fgr GalOx (ref. 35 ). Broadening the substrate range of AA5 enzymes goes hand-in-hand with an extension of the sites where peroxide could be generated by these enzymes. Given the prevalence of galactosyl- and hydroxyl-terminated lipids in cell walls, such a local generation of hydrogen peroxide could then be envisaged as occurring at these sites. Thus, the relative efficiency of Cgr AlcOx and Cgl AlcOx, coupled with the fact that they are independent of complex cofactors such as NAD(P)H and FAD, makes them attractive from a biotechnological perspective not only in enhanced biomass degradation but also as ‘green’ catalysts for aerobic alcohol oxidation. General Unless specified otherwise, ultrapure water (resistivity >18.0 megaohm-cm, Barnstead NanoPure Diamond) was used in the preparation of all buffers, substrates and enzyme assays. Pre-packed nickel nitrilotriacetic acid (Ni-NTA) was purchased from GE Healthcare (Little Chalfont, UK). All alcohols used in enzyme kinetics and product analysis were purchased from Sigma-Aldrich (St Louis, MO, USA) at 98% or higher purity. Peroxide contamination in commercial alcohols was determined using Quantofix, a semiquantitative dip-stick test from Sigma-Aldrich. Alcohols found to be contaminated with peroxide were passed through neutral alumina (previously activated by strong heating under flame) and re-tested. The glycosidases EndoH, EndoH f and PNGaseF were purchased from New England Biolabs (Ipswitch, MA, USA), while α-mannosidase was purchased from Sigma-Aldrich. Proteomics-grade trypsin was purchased from Promega (Madison, WI, USA). Galactose 6-oxidase from F. graminearum was expressed in P. pastoris (Invitrogen, Groningen, the Netherlands) and purified using pre-packed Ni-NTA [29] . Bovine serum albumin and pre-cast 4–20% SDS–PAGE TGX were purchased from Bio-Rad (Hercules, CA, USA). Sequence alignment and phylogenetic analysis The gene models of locus GLRG_05590.1 of C. graminicola M1.001 (encoding UniProt E3QHV8; GenBank EFQ30446) and locus CGGC5_13025 of C. gloeosporioides Nara gc5 (encoding GenBank ELA25906) were downloaded from their respective genome databases [31] , [32] , [33] (accessible via http://www.colletotrichum.org/genomics/ ) and translated to the corresponding protein sequences, herein referred to as Cgr AlcOx and Cgl AlcOx, respectively. Seventy-three other amino-acid sequences of fungal AA5 members, from both subfamily 1 (AA5_2) and subfamily 2 (AA5_2), were extracted from the public version of the CAZy database ( http://www.cazy.org/AA5.html , ref. 16 ). Where present, signal sequences and additional modules, such as carbohydrate-binding modules, were removed to isolate the catalytic modules for bioinformatics analysis. A multiple sequence alignment was produced using Muscle [52] . A distance matrix based on maximum likelihood was then produced using the BLOSUM62 substitution matrix [53] and transformed into a phylogenetic tree using BioNJ [54] . Subfamilies were inferred with the assistance of Secator [55] , and the tree was formatted using Dendroscope [56] . DNA cloning and strain production cDNA encoding Cgr AlcOx without the predicted native signal peptide (MPTLRSALRNLPAALLALAAACEA) [57] , and including a C-terminal His 6 tag-encoding sequence, was commercially synthesized (BioBasic, Markham, Canada), cloned into pUC57 and subcloned into the P. pastoris expression vector pPICZα-C (Invitrogen) flush with the sequence encoding the S. cerevisiae α-factor secretion signal peptide ( Supplementary Table 1 and Supplementary Fig. 1 ). The CgrAlcOx gene was first amplified with PCR using CgrAlcOx-f and CgrAlcOx-r primers ( Supplementary Table 1 ), 0.2 mM dNTPs and Q5 high-fidelity DNA polymerase (New England Biolabs) with supplied buffers. The 1.7-kb PCR product was purified using a commercial anion exchange column (OMEGA Bio-tek). The purified PCR product and pPICZα-C vector were separately digested using XhoI and NotI restriction enzymes for 1 h at 37 °C, and then purified using an ion exchange column. The digested products were combined in a 2:1 insert to vector ratio and ligated using T4 DNA ligase (Lucigen, Middleton, WI, USA) for 2 h at 20 °C. The ligated product was directly transformed into chemically competent E. cloni 10G (Lucigen) using the heat-shock method. cDNA encoding CglAlcOx without the predicted native signal peptide (MVTLYSPFGSLPVALLALAALCEA) [57] , and including a C-terminal His 10 tag-encoding sequence, was commercially synthesized in a codon-optimized form (Genescript, Piscataway, NJ, USA), cloned directly into pPICZα-A using the EcoRI and XbaI restriction sites flush with the sequence encoding the S. cerevisiae α-factor signal peptide, and transformed into chemically competent E. coli DH5α by heat shock. In both cases, transformants were grown overnight at 37 °C on Luria-Bertani-Low-Salt (LBLS) agar plate and selected against 25 μg ml −1 Zeocin (Invitrogen). Surviving colonies were picked and grown overnight at 37 °C in 5 ml LBLS medium with 25 μg ml −1 Zeocin. Plasmids from the overnight cultures were extracted using a commercial miniprep-kit (Geneaid, New Taipei City, Taiwan). The presence of the pPICZα-C-CgrAlcOx and pPICZα-A-CglAlcOx constructs in positive clones was checked by agarose (1%; w/v) gel electrophoresis and the correct insertion of both AlcOx genes into the corresponding vectors was verified by DNA sequencing. Transformations of pCgrAlcOx and pCglAlcOx into P. pastoris X33 were initiated by digesting 2 and 11 μg of plasmid DNA for 1 h at 37 °C with SacI and PmeI (New England Biolabs), respectively. The linearized plasmids were purified using an ion exchange column (Geneaid). The digested plasmids were transformed into electrocompetent P. pastoris X33 cells prepared on the same day [58] . Transformants were grown on YPDS agar plates for 3 days at 30 °C and selected against 100 μg ml −1 Zeocin. Several colonies were streaked on YPDS agar plates increasing Zeocin concentration (250, 500, 750 and 1000 μg ml −1 ) and grown during 3 days at 30 °C to select clones with multicopy insertions. Four colonies from each pCgAlcOx transformation selected from 500 or 1,000 μg ml −1 Zeocin plates were inoculated into 50-ml sterile conical tubes containing 5 ml of BMGY grown in a shaking incubator overnight at 30 °C and 220 r.p.m. Cells were then pelleted by centrifugation at 1,500 g for 5 min, and the BMGY was decanted and replaced with 5 ml of BMMY with 1% ( v/v ) methanol. The culture was shaken at 200 r.p.m. overnight at 18 °C. Regular feeding of 1% methanol every 24 h over 3 days was performed to ensure continuing protein expression. Proteins exported to the liquid medium, via targeting by the S. cerevisiae α-factor signal peptide and cleavage by the P. pastoris Kex 2 enzyme, were separated from cells and solid particulates by centrifugation at 3,000 g for 15 min. Protein production was analysed using SDS–PAGE, and the clone that yielded the highest amount of protein was retained for large-scale production. Site-directed mutagenesis Loop and point variants of Cgr AlcOx were generated using the QuikChange-II Site-directed Mutagenesis kit (Agilent Technologies) according to the supplier’s protocol. The sequences of sense/antisense mutagenic primer pairs and the associated nucleotide replacement are listed in Supplementary Table 1 . The PCR products were treated with 10 units DpnI at 37 °C for 1 h and transformed into the competent E. coli DH5α using the heat-shock method. Positive transformants were selected by plating on LBLS agar plates containing 25 μg ml −1 Zeocin at 37 °C overnight. Plasmids containing the correct mutation were identified using DNA sequencing. Then, the mutant plasmids were linearized with PmeI and transformed into P. pastoris X33 by electroporation, and positive transformants were selected as described above. Large-scale protein production in a shake flask Single colonies of P. pastoris X33 expressing AlcOx variants were individually streaked on agar plate containing 100 μg ml −1 of Zeocin and grown for 2 days at 30 °C. A single colony of each was then picked and inoculated in 10 ml of BMGY at 30 °C shaken at 200 r.p.m. for 8 h. Biomass production was initiated by addition of the 10 ml culture to 1 l of BMGY medium in a 4-l baffled flask with a foam cap shaken at 30 °C during 18–20 h. Cells were harvested by centrifugation at 1,500 g for 5 min under sterile conditions. The cells were quickly resuspended in 1 l of BMMY containing 1% methanol and transferred to sterile 4-l baffled flask with a foam cap. The culture was shaken at 200 r.p.m. overnight at 16 °C. Regular feeding of 1% methanol every 24 h was performed to ensure continuing protein expression. After 3 days of methanol induction, proteins exported to the liquid medium were separated from cells and solid particulates by centrifugation at 3,000 g during 15 min. The supernatant was quickly decanted and stored at 4 °C or used for subsequent purification. Protein purification Liquid medium containing Cgr AlcOx or Cgl AlcOx was first raised to pH 7.5 from 6.0 by dropwise addition of 5 M KOH while slowly stirring. The medium was allowed to equilibrate at 4 °C for 6–18 h, followed by removal of solids by filtration through a sterile 0.45-μm polyethersulfone membrane (Nalgene, New York, NY, USA) that was previously rinsed with ultrapure H 2 O. Purifications were initiated by passing the filtrate through a 5-ml pre-packed Ni-NTA column, pre-equilibrated with 50 mM sodium phosphate buffer at pH 7.5 with 300 mM NaCl at 2 ml min −1 . The column was washed with 70 ml of equilibration buffer (14 column volumes) at 2 ml min −1 and 10 ml of equilibration buffer with 25 mM imidazole at 2 ml min −1 . Proteins were eluted with a linear gradient from 5 to 95% of 500 mM imidazole in 50 mM sodium phosphate buffer at pH 7.5 with 300 mM NaCl at 2 ml min −1 . The total elution volume was 120 ml, which was collected in 1-ml fractions. Both Cgr AlcOx and Cgl AlcOx were eluted at ∼ 90 mM imidazole. Further purification and desalting of Cgr AlcOx and Cgl AlcOx were performed using size exclusion chromatography. Each time, an aliquot of 1–2 ml (4–6 mg ml −1 ) of Ni-NTA-purified AlcOx was loaded on a 16 mm × 600 mm column of Superdex 75 pre-equilibrated with 50 mM sodium phosphate at pH 7.0 at 1 ml min −1 . A total volume of 200 ml of equilibration buffer was applied through the column at 1 ml min −1 . The AlcOxs eluted at ca. 150 ml. SDS–PAGE was performed using pre-cast 4–20% (w/v) polyacrylamide gel in the presence of 2% (w/v) SDS under reducing conditions; proteins were visualized with Coomassie blue R-250 or InVision His-tag In-gel Stain (Life Technologies, Carlsbad, CA, USA; Supplementary Fig. 2 ). The identities of the purified proteins were confirmed using tandem mass spectrometry following in-gel tryptic digests at the Proteomics Core Facility at the University of British Columbia using standard techniques. Protein concentrations of Cgr AlcOx ( ɛ =101,215 M −1 cm −1 ) and Cgl AlcOx ( ɛ =95,715 M −1 cm −1 ) were determined by measuring A 280 ; extinction coefficients were calculated using the ProtParam tool on the ExPASy server ( http://web.expasy.org/protparam/ ). Analytical protein deglycosylation The presence of protein glycosylation on Cgr AlcOx and Cgl AlcOx was determined by treatment with endoglycosidase H from S. plicatus (EndoH, New England Biolabs), endoglycosidase H f (a recombinant protein fusion of Endo H and maltose-binding protein, New England Biolabs), N-glycosidase F from Flavobacterium meningosepticum (PNGaseF, New England Biolabs) or α-mannosidase from Canavalia ensiformis (Sigma-Aldrich). Deglycosylation experiments under denaturing conditions were initiated by adding 20 μg of each protein to denaturing buffer (supplied by the manufacturer) and heating to 100 °C for 10 min, after which samples were diluted to a final volume of 20 μl with 2 μl of 0.5 M sodium phosphate at pH 7.5 or 0.5 M sodium citrate at pH 5.5 for PNGaseF and EndoH/EndoH f , respectively. Finally, 1 μl of either EndoH/EndoH f or PNGaseF was added, and the samples were incubated for 1 h at 37 °C. For PNGaseF, the reaction required 1% tergitol-type NP-40 for deglycosylation activity [59] . Deglycosylation under non-denaturing conditions with α-mannosidase was performed by adding 0.1 U of this enzyme to 20 μg of AA5 AlcOx in 50 mM sodium citrate at pH 5.5. The reaction was incubated overnight at 23 °C. Changes in protein mobility were analysed with SDS–PAGE, followed by staining for protein with Coomassie blue R-250 or carbohydrate with periodic acid-Schiff using a SIGMA Glycoprotein Staining Kit, according to the manufacturer’s protocol ( Supplementary Fig. 2 ). pH profile and temperature stability To determine enzyme activity across a range of pH values, two sets of stock Britton–Robinson buffers [60] were made; each contained 30 mM citrate, phosphate and borate at pH 4.5 and 12. The low and high pH buffer sets were mixed in different proportions to obtain the desired pH values. The final concentration of buffer in the enzyme assay was 17 mM of citrate, phosphate and borate. Enzyme activity was measured using the HRP—2,2'-azino-bis(3-ethylbenzthiazoline-6-sulphonic acid (ABTS)-coupled assay described below with 30 mM of 1-butanol. Temperature stabilities of AA5 AlcOx enzymes were performed by diluting concentrated stock protein into 50 mM sodium phosphate buffer at pH 7.0 to achieve a final protein concentration of 0.35 μg ml −1 . The diluted protein was then heated using a thermocycler at 37, 42, 46 and 51 °C. Samples of protein were taken out at different time intervals, and the activity was measured using the coupled HRP–ABTS assay described below with 30 mM of 1-butanol as the substrate. Initial rate kinetics The kinetics of enzymatic oxidation of alcohols were followed using a colorimetric HRP–ABTS-coupled assay. Oxidation of alcohols to the corresponding aldehyde by AA5 enzymes consumes 1 equivalent of O 2 and generates 1 equivalent of H 2 O 2 ; HRP catalyses the oxidation of ABTS to ABTS ox ( λ max =414 nm, ɛ =36 000 M −1 cm −1 ) using H 2 O 2 . The standard assay routinely used for Fgr GalOx from AA5 (ref. 29 ) was optimized for sensitivity and linearity (see Supplementary Methods ) to contain 50 mM sodium phosphate at pH 8.0, 0.49 mM ABTS, 2.3 μM horseradish peroxidase, 30 mM alcohol and 1.14 pM purified Cgr AlcOx or 0.66 pM purified Cgl AlcOx (assay temperature 23 °C). Under these conditions, formation of ABTS ox gives a linear response between 1 and 4 min that was used to derive initial rates at a range of substrate concentrations for the determination of K m and k cat values. One unit of AlcOx activity was defined as the amount of enzyme necessary for the oxidation of 2 μmol of ABTS per minute, corresponding to the consumption of 1 μmol of O 2 per minute. Enzyme product analysis using 1 H-NMR AA5 AlcOx oxidation products of 1-butanol, glycerol, 2-methyl-1-butanol, benzyl alcohol, cinnamyl alcohol and 2,4-hexa-( E,E )-dien-1-ol were determined using 1 H-NMR. Oxidation of these alcohols was initiated by addition of 45 U of Cgr AlcOx or Cgl AlcOx to a 10-ml solution of 5–90 mM alcohol (5–10 mM for 2,4-hexadien-1-ol), 50 mM sodium phosphate at pH 8.0 and 15 000 U of catalase. Solutions were shaken at 200 r.p.m. for 16 h at 23 °C. In parallel, a reaction without the enzyme was performed as a negative control. Remaining starting materials and products were extracted by addition of 1 ml of deuterated chloroform (CDCl 3 ) to the reaction mixture in a separatory funnel (glycerol oxidation was directly analysed in 80% D 2 O buffer). Products extracted with CDCl 3 were dried with anhydrous sodium sulfate and immediately analysed using a 300-MHz 1 H-NMR spectrometer (Bruker). Electron paramagnetic resonance Pure AA5 AlcOx enzymes were incubated with 1 mM EDTA at 4 °C to remove any weakly bound Cu. After 16 h, EDTA was removed by buffer exchange and the enzyme was concentrated to 0.2 mM in 20 mM 3-morpholinopropane-1-sulfonic acid (MOPS), pH 7.0. Residual tightly bound copper was still present in the sample, and the Cu site occupancy determined by EPR spin quantitation against a standard solution of CuCl 2 ·2H 2 O was 90±10%, where the protein concentration was determined using the Bradford assay. Continuous-wave X-band-frozen-solution EPR spectra of individual samples of Cgr AlcOx and Cgl AlcOx were collected with and without the addition of 10% v/v glycerol (glycerol did not perturb the spectrum) on a Bruker EMX spectrometer operating at 155 K and 9.3 GHz. Spectral simulation was carried out using the Easyspin 4.0.0 software. To investigate redox properties, samples of Cgr AlcOx were incubated with 20 equivalents of sodium dithionite under N 2 atmosphere or 20 equivalents of potassium ferricyanide in air for 1 h, with EPR spectra collected before the addition, after 10 min and after 1 h of incubation. Raw data files in support of this work can be accessed via the library at the University of York ( DOI:10.15124/d1278660-b889-4932-8430-401884176d75 ). Crystallography of Cgr AlcOx Before crystallization, 5 mg of purified Cgr AlcOx were incubated with 10 μl of EndoH f (New England Biolabs) in a total volume of 5 ml in 50 mM phosphate buffer, pH 7.5 for 2 h at 20 °C to reduce sample complexity because of N-glycosylation. The sample was then loaded on to a 1-ml Histrap HP column (GE Healthcare), previously equilibrated in the same incubation buffer. EndoH f was recovered in the flow-through while Cgr AlcOx was eluted with a linear gradient of 0–500 mM imidazole in the same buffer. Cgr AlcOx was buffer-exchanged to 20 mM MOPS, pH 7.0 and concentrated up to 8 mg ml −1 in a 0.5-ml Amicon centrifugal filter (Millipore). Carbohydrate cleavage was confirmed by an ∼ 8-kDa difference (compared with the native protein) in a 12% SDS–PAGE gel. Crystallization trials were set up with the vapour diffusion sitting-drop technique using a Mosquito robot (TTP Labtech, Melbourn, UK). Apo-protein crystals of hexagonal appearance were obtained after optimization and microseeding in a condition composed of 0.1 M imidazole, pH 8.0, 12% v/v polyethylene glycol 8.000 and 4.5% 1-butanol. Crystals were soaked in mother liquor supplemented with 40% v/v 2-methyl-2,4-pentanediol, followed by fast-freezing in liquid nitrogen. Diffraction data ( Table 2 ) were collected at the Diamond Light Source (UK), beamline I04, at a wavelength of 0.979 Å. Table 2 Data collection and refinement statistics (molecular replacement). Full size table Crystals of the protein, in complex with copper, and of tetragonal appearance were obtained after optimization and microseeding in 50% tacsimate buffer (Hampton Research, Aliso Viejo, CA, USA), at pH 6.5, followed by soaking. The crystal was soaked in a solution of 52% tacsimate buffer, pH 6.0, with the addition of copper sulfate powder to the drop. After 15 days, the crystals were harvested using 52% tacsimate buffer, pH 6.5, 25% ( v/v ) ethylene glycol as cryoprotectant and immediately fast-frozen in liquid nitrogen. Diffraction data ( Table 2 ) were collected at the Diamond Light Source, beamline I03, at a wavelength of 0.979 Å. Structure solution and refinement All diffraction data were indexed, integrated and scaled with XDS [61] , and the following processing steps were performed with the CCP4i software suite [62] . Molecular replacement was performed with MOLREP [63] using the protein atoms only, from the two conserved domains, of F. graminearum galactose 6-oxidase as the model (2EIE (ref. 35 )). Cgr AlcOx shares 47% identity with the two domains of this model (that is, excluding the CBM32 of Fgr GalOx). The structure was rebuilt and refined with COOT [64] and REFMAC5 (ref. 65 ). The two Asn-linked N -acetylglucosamine residues remaining from the deglycosylation step were validated with Privateer [66] . An anomalous map was built to confirm the heavy atom nature of the positive density localized in the active centre (Cu, consistent with the EPR spectra, vide supra ). For the apo-protein, 0.5% of Ramachandran outliers were detected and 94.6% of the amino acids were in the preferred region. In the case of the copper-containing crystal, 0.42% of Ramachandran outliers were detected and 95.2% of the amino acids were in the preferred regions. Structural figures were made using CCP4 mg (ref. 67 ). Accession codes: Crystallographic structures of apo- Cgr AlcOx and Cu- Cgr AlcOx have been deposited in the Research Collaboratory for Structural Bioinformatics Protein Data Bank under PDB ID 5C86 and 5C92 , respectively. How to cite this article: Yin, D. L. et al. Structure–function characterization reveals new catalytic diversity in the galactose oxidase and glyoxal oxidase family. Nat. Commun. 6:10197 doi: 10.1038/ncomms10197 (2015).